Cobalt(III)-catalyzed asymmetric ring-opening of 7-oxabenzonorbornadienes via indole C–H functionalization Asymmetric ring-opening of 7-oxabenzonorbornadienes is achieved via Co-catalyzed indole C–H functionalization. The utilization of chiral Co-catalyst consisting of a binaphthyl-derived trisubstituted cyclopentadienyl ligand resulted in high yields (up to 99%) and excellent enantioselectivity (>99% ee) for the target products with tolerance for diverse functional groups. Opposite diastereoselectivities are obtained with chiral Co-catalyst or Cp*CoI 2 CO. Combined experimental and computational studies suggest β -oxygen elimination being the selectivity-determining step of the reaction. Meanwhile, the reactions of 7-azabenzonorbornadiene could also be executed in a diastereodivergent manner. Tremendous developments have been achieved in the past decades for transition-metal-catalyzed C–H functionalization reactions [1] , [2] , [3] , [4] , [5] , [6] , [7] , [8] . Recently, exploring 3d metal complexes in C–H functionalization has attracted considerable attention because of the earth-abundance and low toxicity of these metals compared with the 4d and 5d counterparts [9] , [10] , [11] , [12] . Pioneered by the groups of Matsunaga and Kanai [13] , [14] , Ackermann [15] , Ellman [16] , Glorius [17] , and Chang [18] , cyclopentadienyl (Cp)-Co complexes have been identified as competent catalysts for various C–H functionalization reactions, which often exhibit complementary reactivity and selectivity to those with Cp-Rh catalysts [14] , [18] , [19] , [20] , [21] , [22] , [23] , [24] , [25] , [26] . Particularly, the Cp-Co complexes derived from a chiral Cp ligand [27] , [28] , [29] or achiral Cp ligand in combination with chiral counteranions [30] , [31] , [32] , [33] , [34] , [35] , [36] , [37] were demonstrated suitable for asymmetric C–H functionalization reactions (Fig. 1a ) [12] . In this regard, the groups of Ackermann [30] , Matsunaga [31] , [32] , [33] , [34] , Cramer [27] , [28] , [29] , and Shi [35] , [36] , [37] independently reported Co-catalyzed asymmetric aryl C–H functionalization with unactivated olefins, maleimides or dioxazolones. Previously, the modifications of the Cp ring have resulted in an extensive array of Cp-metal catalysts [38] , [39] , [40] , [41] , [42] , [43] , [44] . However, whether the use of chiral Cp ligands in Co-catalyzed C–H functionalization reactions can influence the reaction outcomes of beyond enantioselectivity remains underdeveloped [13] , [27] , [28] , [29] , [45] , [46] . Fig. 1: Asymmetric ring-opening of bicyclic olefins via Co-catalyzed C–H functionalization. a Co catalyzed asymmetric C–H functionalization. b Common mechanistic manifold of asymmetric ring-opening of bicyclic alkenes. c Co-catalyzed asymmetric ring-opening of 7-oxabenzonorbornadienes (this work). Full size image Asymmetric ring-opening (ARO) of strained bicyclic olefins is an important platform for building-up molecular complexity (Fig. 1b ) [47] , [48] , [49] . Merging ARO reactions with transition-metal-catalyzed C–H activation has become an area of recent interest [50] , [51] , [52] , [53] , [54] , [55] , [56] , [57] , [58] , [59] , [60] . In this regard, the groups of Zheng and Li [53] , and Cramer [54] independently reported the ARO reactions of 7-azabenzonorbornadienes and other aza-bicyclic olefins under Rh-catalysis, in which β- nitrogen elimination was a key step. However, to the best of our knowledge, the C–H activation-induced ARO reactions of 7-oxabenzonorbornadienes via β- oxygen elimination remained elusive, probably due to the competitive dehydration [61] , [62] or direct reductive elimination [63] , [64] as a side reaction pathway. Mechanistically, it was regarded that the ARO reactions proceeded via the exo -coordination of a carbon–metal species to the olefin moiety, migratory insertion and cis - β -heteroatom elimination [47] , [53] , [54] , [55] , [56] , [57] , [58] , [59] , [60] . And the migratory insertion was speculated as the enantioselectivity-determining step in the ARO reactions (Fig. 1b ) [47] , [53] , [54] . In line with our continuous interest in developing transition-metal-catalyzed asymmetric C–H functionalization reactions [65] , [66] , [67] , [68] , [69] , [70] , [71] , we envisioned that asymmetric indole C–H functionalization with 7-oxabenzonorbornadienes might be accomplished by using a chiral Cp-Co catalyst [56] (Fig. 1c ). In this work, high yields and excellent stereoselectivity were obtained for a wide range of cis- ring-opening products under the optimal conditions. More interestingly, the utilization of Cp*Co(CO)I 2 as the catalyst led to reversed diastereoselectivities favoring the trans -ring-opening products. The misassigned relative configuration of the products in the previous literature was corrected accordingly [56] . Combined experimental and computational studies suggested the mechanistic pictures of the CpCo-catalyzed ARO reactions where cis - and trans - β -oxygen elimination work as the selectivity-determining step for enantioselective and racemic reactions, respectively. Such results are different from the previous cognition [47] , [53] , [54] , [55] , [56] , [57] , [58] , [59] , [60] , [61] , [62] , [63] , [64] . As an extension, 7-azabenzonorbornadiene could also be applied in the similar ARO reactions in a diastereodivergent manner. Herein, we report the results from this study. 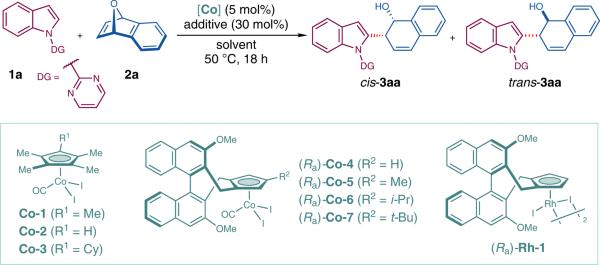Table 1 Optimization of reaction conditionsa No description available Reaction development Our study commenced with the optimization of the reaction conditions using N -pyrimidinylindole ( 1a , 0.05 mmol) and 7-oxabenzonorbornadiene ( 2a , 1.5 equiv) as model substrates (Table 1 ). When achiral catalyst Cp*CoI 2 CO ( Co-1 , 5 mol%) and CsOAc (30 mol%) were utilized, the reaction proceeded smoothly in trifluoroethanol (TFE, 0.3 mL) at 50 °C, leading to the designed ring-opening product 3aa as a mixture of cis and trans isomers (10:90 dr) in a combined yield of 95% (entry 1). Variating the substituent of the Cp ring of the catalyst ( Co-2 and Co-3 , R 1 = H and Cy) did not provide better yields or ratio of cis - 3aa / trans - 3aa (entries 2 and 3). On the contrary, when the chiral Co-complexes consisting of a chiral binaphthyl-derived Cp ligand [( R a )- Co-4 –( R a )- Co-7 ] were used, the diastereoselectivity of the reaction was reversed, with cis - 3aa being the major product (entries 4–7). As the substituent of the Cp ring became bulkier (R 2 = H, Me, i -Pr and t -Bu), both the ratio of cis - 3aa / trans - 3aa (80:20–95:5 dr) and the ee of cis - 3aa (69 to >99%) increased steadily albeit with moderate combined yield of 3aa (10–25%). It was found that the reaction efficiency could be significantly influenced by the additive and solvent. Replacing CsOAc to CsOPiv, NaOPiv or HOPiv resulted in the elevated combined yields of cis- 3aa (39–60%), high diastereoselectivity (up to 96:4 dr) and superior enantioselectivity (>99% ee), with NaOPiv as the best choice among tested (entries 8–10). Switching the solvent to MeOH, DCM or toluene totally shutdown the reaction. However, the utilization of hexafluoroisopropanol (HFIP) led to nearly quantitative formation of cis - 3aa (98% yield) but with slightly decreased dr (93:7) and ee (98%) (entry 11). The stereochemical control could be restored to excellent level by employing mixed solvents of TFE and HFIP (entries 12 and 13). Overall, the optimal reaction outcomes (98% yield, 95:5 dr and >99% ee for cis - 3aa ) were obtained when the ratio of TFE and HFIP (v/v) was set to 3:1 (entry 13). In addition, the reactions between 1a and 2a were conducted under the ( R a )- Rh-1 catalysis (entry 14, also see the Supplementary Information for details) [53] , but both cis - and trans - 3aa were not detected, while 1a and 2a were recovered. These results demonstrated that the Co-catalysts exhibit unique reactivity for the ARO reaction of 7-oxabenzonorbornadiene. Table 1 Optimization of reaction conditions a Full size table With the optimal conditions in hands, the scope of substituted indoles was next investigated (Fig. 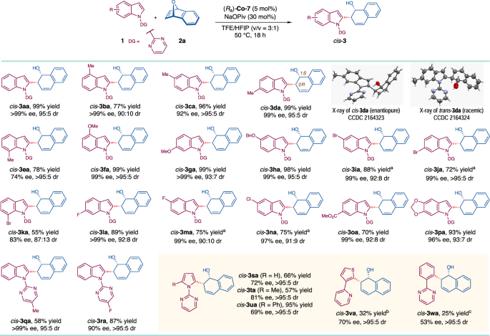Fig. 2: Substrate scope: Indoles and other arenes. Reaction conditions:1(0.10 mmol)2a(0.15 mmol), (Ra)-Co-7(5 mol%), NaOPiv (30 mol%) in TFE/HFIP (0.4 mL, v/v = 3:1) at 50 °C for 18 h. Note: (a) In TFE/HFIP/DCM (0.5 mL, v/v/v = 3:1:1) at 50 °C for 18 h. (b) (Ra)-Co-7(10 mol%), Zn(OAc)2(30 mol%) instead of NaOPiv (30 mol%) was used, in TFE/HFIP (0.4 mL, v/v = 3:1) at 60 °C for 24 h. (c) (Ra)-Co-7(10 mol%), Zn(OAc)2(30 mol%) instead of NaOPiv (30 mol%) was used, in TFE/HFIP (0.4 mL, v/v = 3:1) at 70 °C for 24 h. 2 ). Indoles bearing a methyl group at the C4-, C5- or C6-position were well tolerated. The corresponding products cis - 3ba – 3da were afforded in high yields (77–99%) with good to excellent diastereoselectivity and excellent enantioselectivity (90:10 to >95:5 dr and 92 to >99% ee). However, the reaction of C7-methyl substituted indole became sluggish where the yield and ee value of cis - 3ea were decreased to 78% and 74%, respectively. The influences of other electron-donating groups including methoxy and benzyloxy at the C4-, C5- or C6-position were also investigated. The desired products cis - 3fa – 3 ha were all obtained efficiently (98–99% yields, 93:7 to >95:5 dr, 99 to >99% ee). Furthermore, a variety of electron-deficient indoles bearing halogen substituents (fluoride, chloride and bromide) or an ester group (CO 2 Me) at these positions were well tolerated. In general, good yields (70–88%) and excellent stereochemical control (90:10 to >95:5 dr and 97 to >99% ee) were achieved for the formation of cis - 3ia , 3ja , 3la – 3oa . Notably, introducing a bromide group at the C7-position of the indole ring largely retarded the reaction, leading to cis - 3ka in moderate yield (55%) with lowered stereoselectivity (87:13 dr and 83% ee). The reaction could further accommodate [1,3]dioxolo-substituted indole substrate and variations of the electronic properties of the N -pyrimidinyl directing group ( cis - 3pa – 3ra , 58–93% yields, 93:7 to >95:5 dr and 90 to >99% ee). Pyrrole derivatives also well participated in the reaction and the C2-substituents (methyl or phenyl) did not lead to deleterious effects on the reaction outcomes ( cis - 3sa – 3ua , 57–95% yields, >95:5 dr and 69–81% ee). Moreover, thiophene and benzene derivatives can also be applied in the reactions with 7-oxabenzonorbornadiene, albeit with diminished yields of cis - 3va and cis - 3wa (25–32% yields, >95:5 dr and 53–70% ee) mainly due to recovered substrates 1 v and 1w . Samples of cis - 3da (enantiopure) and trans - 3da (racemic) were subjected to X-ray crystallographic analyses. Their structures, relative configurations, and the absolute configuration of cis - 3da (1 S ,2 R ) were assigned unambiguously. Fig. 2: Substrate scope: Indoles and other arenes. Reaction conditions: 1 (0.10 mmol) 2a (0.15 mmol), ( R a )- Co-7 (5 mol%), NaOPiv (30 mol%) in TFE/HFIP (0.4 mL, v/v = 3:1) at 50 °C for 18 h. Note: (a) In TFE/HFIP/DCM (0.5 mL, v/v/v = 3:1:1) at 50 °C for 18 h. (b) ( R a )- Co-7 (10 mol%), Zn(OAc) 2 (30 mol%) instead of NaOPiv (30 mol%) was used, in TFE/HFIP (0.4 mL, v/v = 3:1) at 60 °C for 24 h. (c) ( R a )- Co-7 (10 mol%), Zn(OAc) 2 (30 mol%) instead of NaOPiv (30 mol%) was used, in TFE/HFIP (0.4 mL, v/v = 3:1) at 70 °C for 24 h. Full size image The reactions of various 7-oxabenzonorbornadiene-derivatives were also considered (Fig. 3 ). Symmetrically disubstituted 7-oxabenzonorbornadienes (2,3-dimethyl, 2,3-dimethoxy, 2,3-difluoro, 2,3-benzo, 1,4-dimethoxy and 1,4-dimethyl) participated in the desired reactions smoothly, giving rise to cis - 3ab , 3ad – 3ag in reasonable yields (50–81%) with good to excellent stereoselectivity (87:13 to >95:5 dr and 94 to >99% ee). To be noted, cis - 3ac was afforded in only 35% yield, but with >95:5 dr and 95% ee. It was postulated that the electron-rich nature of cis - 3ac caused the side reaction of dehydration [61] . Methyl-substituent at two bridge-head positions led to moderate yield (62%) and enantiopurity (52% ee) of cis - 3ah . The reaction of unsymmetrically disubstituted (1,2-dimethyl) substrate generated a pair of regioisomers cis - 3ai (43% yield) and cis - 3ai′ (32% yield), both of which were obtained with excellent diastereo- and enantioselectivity (up to >95:5 dr and >99% ee). Fig. 3: Substrate scope: 7-Oxabenzonorbornadienes. Reaction conditions: 1a (0.10 mmol), 2 (0.15 mmol), ( R a )- Co-7 (5 mol%), NaOPiv (30 mol%) in TFE/HFIP (0.4 mL, v/v = 3:1) at 50 °C for 18 h. Full size image Mechanistic studies In order to understand the origins for the opposite diastereoselectivity with Co-1 (Conditions A) or ( R a )- Co-7 (Conditions B) and for the enantioselectivity in the latter case, a series of mechanistic studies was performed. In a simplified catalytic cycle (Fig. 4a ), the reaction starts with the C–H activation of indole substrate 1a by a Cp-Co complex I (X = OAc or OPiv, L = CO or solvent), which leads to a cyclometallated Co complex II . Deuterium-labeling reactions of 1a were conducted under both conditions using TFE-D 3 or mixed solvents of TFE-D 3 and HFIP-D 2 (v/v = 3:1) (Fig. 4b ). High deuteration ratio at the C2 position of the indole ring was observed in both cases (>95% for Conditions A and 83% for Conditions B), which implied the indole C–H activation step should be reversible. Meanwhile, H/D kinetic isotope effect (KIE) experiments using 1a and 1a-2-D revealed small k H / k D values of 1.1 for Conditions A and 1.3 for Conditions B, respectively (Fig. 4c ). These results suggested that the indole C–H activation was not involved in the turn-over limiting step of the catalytic cycle. Next, Co complex II undergoes ligand exchange with 7-oxabenzonorbornadiene 2a , which generates an olefin-coordinated Co complex III . Starting from this intermediate, there exist two competing reaction pathways, exo - or endo -migratory insertion, leading to cis - IV and trans - IV , respectively. The subsequent C–O bond-cleavage proceeds via the cis - or trans - β -oxygen elimination, which could be assisted by acetic acid generated in the C–H activation step. The catalytic cycle is finally closed by releasing the products cis - 3aa or trans - 3aa with the concomitant regeneration of Co complex I . In addition, 12 C/ 13 C KIE at natural 13 C abundance was determined by quantitative 13 C NMR experiments for the reaction of 1a with 2a catalyzed by ( R a )- Co-7 (3 mmol scale) [72] , [73] . Significant 12 C/ 13 C KIE values were observed for both carbon atoms [1.025(3) and 1.012(3)] of the newly formed C=C double bond of cis - 3aa , suggesting the β -oxygen elimination being the rate-determining step (Fig. 4d ). Fig. 4: Proposed catalytic cycle and deuterium-labeling and kinetic isotope effect experiments. a Proposed catalytic cycle. b Deuterium-labeling reactions of 1a . c H/D Kinetic isotope effect (KIE) experiments. ( d ) 12 C/ 13 C KIE experiments. Full size image DFT calculations were performed for the reactions between 1a and 2a with either Co-1 or ( R a )- Co-7 as the catalyst (Fig. 5 , also see the Supplementary Information and Supplementary Data 1 for details). The calculated energy profiles indicated that the β -oxygen elimination was the rate- and stereoselectivity-determining step in both cases, and thus all the precedent steps were reversible. In the reaction promoted by Co-1 , the energy of the transition state for trans - β -elimination TS- trans - rac was lower than that for the cis - β -elimination transition state TS- cis - rac by 3.2 kcal/mol, which qualitatively reproduced the preferential formation of trans - 3a over cis - 3a . It should be noted that the cis - β -elimination relied on a temporary Co–O coordination bond [B(Co–O) = 2.02 Å] in a cationic transition state TS- cis - rac , while in TS- trans - rac such interaction did not exist and the oxygen atom was located in the opposite side of the original 7-oxabenzonorbornadiene ring. Thus, an additional acetate anion was allowed to coordinate to the Co center in TS- trans - rac , forging a highly charge-separate but overall neutral transition state. The variance on the coordination mode of the Co center in TS- cis - rac and TS- trans - rac was believed to contribute to the calculated energy difference between these two transition states. The situation was changed significantly when ( R a )- Co-7 was employed as the catalyst. The steric congestion around the Co center could not accommodate the coordination of an additional anion to the Co center as in TS- trans - rac , which raised the energetic barrier of the trans - β -oxygen elimination, and thus made the cis - β -oxygen elimination the dominant reaction pathway. In order to shed light on the origin of the asymmetric induction with ( R a )- Co-7 , the key transition states of cis - β -oxygen elimination leading to (1 S ,2 R )- 3aa ( TS- cis - SR , 0.0 kcal/mol) and (1 R ,2 S )- 3aa ( TS- cis - RS , 8.1 kcal/mol), respectively, were located. The large energy difference between these two transition states was in well accordance with the exceedingly high enantioselectivity (>99% ee) observed in the most cases experimentally. The specific substrate orientation in TS- cis - RS induced severe destabilizing structural features including (1) weak coordination of the C2=C3 bond of the indole ring to the Co center [B(Co–C2) = 2.26 Å and B(Co–C3) = 2.62 Å] resulted from the geometric distortion of the substrates compared with that in TS- cis - SR [B(Co–C2) = 2.35 Å and B(Co–C3) = 2.33 Å], and (2) steric repulsion between the substrates and the tert -butyl substituent on the cyclopentadienyl ring in TS- cis - RS , which was exemplified by the short distances between several pairs of hydrogen atoms in the two structural components [B(H a –H d ) = 2.08 Å, B(H b –H e ) = 2.06 Å and B(H c –H e ) = 2.29 Å]. To be noted, some minor effects which cause diminished enantioselectivity for the substrates with certain substitution patterns might not be included in the computational model. Fig. 5: Optimized structures of the transition states for the β -oxygen elimination step. Calculated at the PWPB95-D3(BJ)/def2-TZVPP (SMD, TFE)//B3LYP-D3(BJ)/def2-SVP (gas) level of theory. The relative Gibbs free energies (Δ G sol ) are in kcal/mol. The distances of forming/cleaving bonds are in Å. Full size image Synthetic Applications As an extension, N -Boc 7-azabenzonorbornadiene 6 was also investigated in this chiral Cp-Co catalyzed ARO reactions (Fig. 6 , see the Supplementary Information for details). In the presence of ( S a )- Co-4 as the catalyst, AgSbF 6 , Zn(OAc) 2 , as the additives, and TFE as the solvent, the cis -ring-opening products ( cis - 7aa – 7ae ) were delivered in morderate yields (55-63%) with excellent stereoselectivity (92:8 to 95:5 dr, 94–96% ee). More interestingly, when the solvent was changed to toluene, the ring-opening products with the opposite relative configuration ( trans - 7aa – 7ae ) were obtained in promising results (51–57% yields, 93:7 to >95:5 dr, 63–86% ee). Besides, the reactions of N -tosyl 7-azabenzonorbornadiene could also be executed in a diastereodivergent manner, giving the cis - 7af / trans - 7af in morderate yields (44–50%) with moderate to good stereoselectivity (95:5 to >95:5 dr, 63–91% ee). Unfortunatly, when 7-oxabenzonorbornadiene 2a was subjected to the conditions for the synthesis of trans - 7 , only the dehydration product was delivered in almost quantitative yield [61] , [62] . Fig. 6: ARO reactions of 7-azabenzonorbornadiene. Reaction conditions A: 1 (0.15 mmol), 6 (0.10 mmol), ( S a )- Co-4 (10 mol%), AgSbF 6 (20 mol%), Zn(OAc) 2 (50 mol %) in TFE (1.0 mL) at 80 °C for 48 h. Reaction conditions B: 1 (0.15 mmol), 6 (0.10 mmol), ( S a )- Co-4 (10 mol%), AgNTf 2 (20 mol%), Fe(OAc) 2 (50 mol%) in toluene (1.0 mL) at 70 °C for 48 h. Full size image The Co-catalyzed indole C–H functionalization/asymmetric ring-opening of 7-oxabenzonorbornadienes could be performed on a gram-scale. The reaction between 1a (3.0 mmol) and 2a (4.5 mmol) proceeded well in the presence of a lowered loading of ( R a )- Co-7 (2.5 mol%), delivering cis - 3aa in 97% yield (989.4 mg) with 95:5 dr and 98% ee after 48 h (Fig. 7a ). Besides, cis - 3aa and cis - 3ia underwent hydrogenation and Suzuki–Miyaura cross-coupling reactions, respectively, generating the corresponding products 4 and 5 in good yields (95% and 85%) without the erosion of enantiopurity (Figs. 7 b, 7c ). In addition, the N -Boc protecting group of trans - 7ab could be readily removed in the presence of hydrogen chloride (Fig. 7d ), and the further transformation to trans - 7ab′ unambiguously assigned their absolute configuration (Fig. 7e ). Fig. 7: Gram-scale reaction and product transformations. Reaction conditions: (a) 1a (3.0 mmol), 2a (4.5 mmol), NaOPiv · H 2 O (0.9 mmol), ( R a )- Co-7 (0.075 mmol), TFE/HFIP (12.0 mL, v/v = 3:1), 50 °C, 48 h. (b) Pd/C (0.1 equiv), H 2 (1 atm), EtOAc (0.1 M), rt., 24 h. (c) PhB(OH) 2 (2.0 equiv), Pd 2 dba 3 (2.5 mol%), SPhos (10 mol%), Na 2 CO 3 (0.5 equiv), toluene/EtOH/H 2 O (1.25 mL, v/v/v = 3:1:1). (d) HCl (2.0 mL, 4 M in dioxane), rt., overnight. (e) DMAP (1.0 equiv), TsCl (1.2 equiv), Et 3 N (6.0 equiv), DCM (2.0 mL), rt., 12 h. Full size image In conclusion, we have developed Co-catalyzed ARO reactions of 7-oxabenzonorbornadienes via indole C–H activation. The reactions demonstrated opposite diastereoselectivity with binaphthyl-derived chiral cyclopentadienyl-derived cobalt catalysts when compared with that using Cp*Co(CO)I 2 . Good yields and excellent enantioselectivity were obtained for a wide range of substrates. 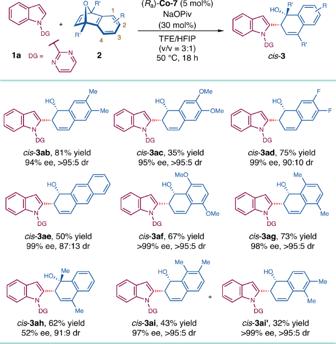Fig. 3: Substrate scope: 7-Oxabenzonorbornadienes. Reaction conditions:1a(0.10 mmol),2(0.15 mmol), (Ra)-Co-7(5 mol%), NaOPiv (30 mol%) in TFE/HFIP (0.4 mL, v/v = 3:1) at 50 °C for 18 h. Combined experimental and computational studies offered deep mechanistic insights into the reaction profile and the origins of the diastereo- and enantioselectivity. Moreover, the Co-catalyzed ARO reactions of 7-azabenzonorbornadiene were also realized in a diastereodivergent manner. 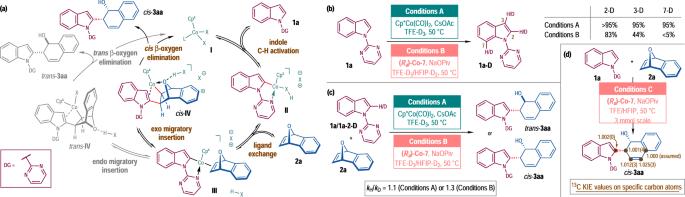Fig. 4: Proposed catalytic cycle and deuterium-labeling and kinetic isotope effect experiments. aProposed catalytic cycle.bDeuterium-labeling reactions of1a.cH/D Kinetic isotope effect (KIE) experiments. (d)12C/13C KIE experiments. General procedure for the enantioselective synthesis of cis- 3 A sealed tube with a magnetic stir bar was charged with ( R a )- Co-7 (4.0 mg, 0.005 mmol), NaOPiv · H 2 O (4.4 mg, 0.03 mmol), 1 (0.1 mmol), 2 (0.15 mmol), TFE (0.3 mL) and HFIP (0.1 mL) under argon atmosphere. The mixture was stirred at 50 °C for 18 h. Afterwards, the mixture was cooled to room temperature and quenched by saturated NH 4 Cl aqueous solution (20 mL). The resulted mixture was extracted with ethyl acetate (3 × 15 mL). The combined organic phase was dried over anhydrous Na 2 SO 4 and filtered. 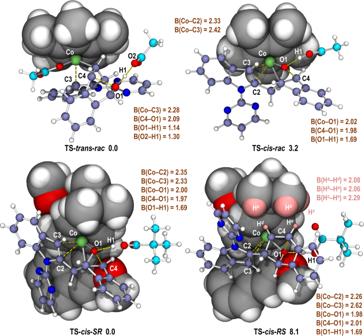Fig. 5: Optimized structures of the transition states for theβ-oxygen elimination step. Calculated at the PWPB95-D3(BJ)/def2-TZVPP (SMD, TFE)//B3LYP-D3(BJ)/def2-SVP (gas) level of theory. The relative Gibbs free energies (ΔGsol) are in kcal/mol. The distances of forming/cleaving bonds are in Å. All the volatiles were evaporated under reduced pressure. The remaining residue was purified by column chromatography on silica gel (hexanes/ethyl acetate = 8:1 to 4:1) to afford cis - 3 . General procedure for the enantioselective synthesis of cis- 7 A sealed tube with a magnetic stir bar was charged with ( S a )- Co-4 (7.6 mg, 0.010 mmol), AgSbF 6 (6.8 mg, 0.020 mmol), Zn(OAc) 2 (9.2 mg, 0.050 mmol), 1 (0.15 mmol), 6 (24.3 mg, 0.10 mmol) and TFE (1.0 mL) under argon atmosphere. The mixture was stirred at 80 °C for 48 h. Then, the mixture was cooled to room temperature and quenched by saturated NH 4 Cl aqueous solution (20 mL). The resulted mixture was extracted with ethyl acetate (3 × 15 mL). The combined organic phase was dried over anhydrous Na 2 SO 4 and filtered. All the volatiles were evaporated under reduced pressure. The remaining residue was purified by column chromatography on silica gel (hexanes/ethyl acetate = 10:1 to 6:1) to afford cis - 7 . General procedure for the enantioselective synthesis of trans- 7 A sealed tube with a magnetic stir bar was charged with ( S a )- Co-4 (7.6 mg, 0.010 mmol), AgNTf 2 (7.8 mg, 0.020 mmol), Fe(OAc) 2 (8.7 mg, 0.050 mmol), 1 (0.15 mmol), 6 (24.3 mg, 0.10 mmol) and toluene (1.0 mL) under argon atmosphere. The mixture was stirred at 70 °C for 48 h. Afterwards, the mixture was cooled to room temperature and quenched by saturated NH 4 Cl aqueous solution (20 mL). The resulting mixture was extracted with ethyl acetate (3 × 15 mL). The combined organic phase was dried over anhydrous Na 2 SO 4 and filtered. 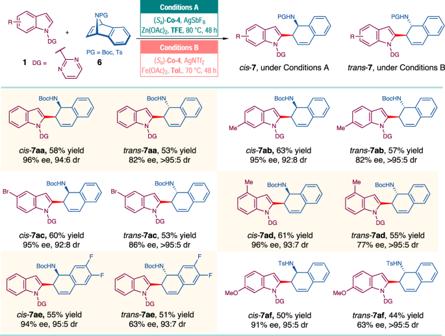Fig. 6: ARO reactions of 7-azabenzonorbornadiene. Reaction conditions A:1(0.15 mmol),6(0.10 mmol), (Sa)-Co-4(10 mol%), AgSbF6(20 mol%), Zn(OAc)2(50 mol %) in TFE (1.0 mL) at 80 °C for 48 h. Reaction conditions B:1(0.15 mmol),6(0.10 mmol), (Sa)-Co-4(10 mol%), AgNTf2(20 mol%), Fe(OAc)2(50 mol%) in toluene (1.0 mL) at 70 °C for 48 h. 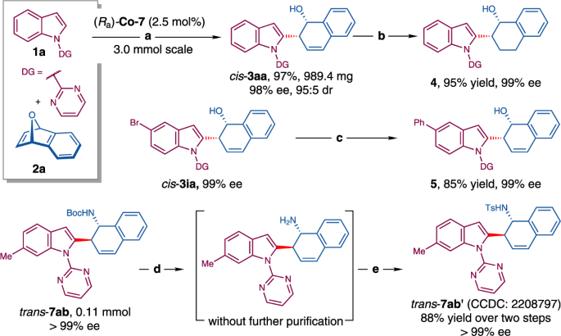Fig. 7: Gram-scale reaction and product transformations. Reaction conditions: (a)1a(3.0 mmol),2a(4.5 mmol), NaOPiv · H2O (0.9 mmol), (Ra)-Co-7(0.075 mmol), TFE/HFIP (12.0 mL, v/v = 3:1), 50 °C, 48 h. (b) Pd/C (0.1 equiv), H2(1 atm), EtOAc (0.1 M), rt., 24 h. (c) PhB(OH)2(2.0 equiv), Pd2dba3(2.5 mol%), SPhos (10 mol%), Na2CO3(0.5 equiv), toluene/EtOH/H2O (1.25 mL, v/v/v = 3:1:1). (d) HCl (2.0 mL, 4 M in dioxane), rt., overnight. (e) DMAP (1.0 equiv), TsCl (1.2 equiv), Et3N (6.0 equiv), DCM (2.0 mL), rt., 12 h. All the volatiles were evaporated under reduced pressure. The remaining residue was purified by column chromatography on silica gel (hexanes/ethyl acetate = 10:1 to 6:1) to afford trans - 7 .